Subduction of fracture zones controls mantle melting and geochemical signature above slabs For some volcanic arcs, the geochemistry of volcanic rocks erupting above subducted oceanic fracture zones is consistent with higher than normal fluid inputs to arc magma sources. Here we use enrichment of boron (B/Zr) in volcanic arc lavas as a proxy to evaluate relative along-strike inputs of slab-derived fluids in the Aleutian, Andean, Cascades and Trans-Mexican arcs. Significant B/Zr spikes coincide with subduction of prominent fracture zones in the relatively cool Aleutian and Andean subduction zones where fracture zone subduction locally enhances fluid introduction beneath volcanic arcs. Geodynamic models of subduction have not previously considered how fracture zones may influence the melt and fluid distribution above slabs. Using high-resolution three-dimensional coupled petrological-thermomechanical numerical simulations of subduction, we show that enhanced production of slab-derived fluids and mantle wedge melts concentrate in areas where fracture zones are subducted, resulting in significant along-arc variability in magma source compositions and processes. Oceanic fracture zones are born where spreading centres are offset, creating strong gradients in oceanic floor age and vertical offsets in the oceanic lithosphere [1] . Whether or not fracture zones are weaker than normal oceanic lithosphere is a subject of debate [2] , [3] , [4] , [5] , [6] . However, several lines of evidence, such as tectonic uplift [4] and localized volcanic activity distributed along fracture zones [5] , suggest that oceanic fracture zones may indeed be zones of weakness. Dynamic models of Pacific fracture zones [6] show that they need to be mechanically weak (yield strength <10 MPa) in order to have synthetic gravity offsets consistent with the observations. Other evidence indicative of fracture zone weakness is the statistically prevalent occurrence of intraplate oceanic earthquakes near fracture zones [7] . In addition, fracture zones provide conduits for seawater infiltration where peridotites locally may be exposed to intense hydrothermal alteration producing serpentinites. Serpentinites have low mechanical strength compared with unaltered peridotite [8] , and laboratory experiments show that, at depths of approximately 30–100 km, serpentine is weaker than most other mantle minerals (for example, pyroxene, plagioclase, and wet and dry olivine [9] ). Deformation experiments show that the presence of a small amount of serpentine (~10%) reduces drastically the strength of an altered peridotite to that of pure serpentinite [8] . Serpentinites are commonly associated with major fracture zones on the Juan de Fuca, Pacific, Cocos and Nazca plates [10] , [11] , [12] , [13] , [14] , and potentially create zones of weakness in the oceanic lithosphere [15] to depths of 20 km or more below the oceanic Moho [16] . There is wide consensus among researchers that slab-derived fluids exert significant influence on partial melting of the mantle wedge beneath volcanic arcs. Moreover, seismic studies are consistent with local addition of up to 2 wt% of slab-derived hydrous fluids to mantle wedge domains [17] . Compared with regions where ‘normal’ oceanic lithosphere is subducted, the presence of fracture zones will likely deliver anomalous volumes [18] of water-rich serpentinite to depths of 100 km or more [19] , and thus augment the flux of slab-derived fluids to the overlying mantle. However, there is no clear view on the effect, if any, of fracture zone subduction on melt distribution below volcanic arcs. As volcanic arc lavas generally carry signals of hydrous fluids, they can be used as probes to assess spatial variations in fluxes of slab-derived components and how these might correlate with along-strike heterogeneities in downgoing subducting plates. There is compelling evidence that compositions of volcanic arc magmas may be strongly influenced by the amount and nature of aqueous fluids released by the subducting plates [20] , [21] , [22] . A variety of geologic and petrologic observations suggest that lateral variations in chemical fluxes and processes of magma generation in volcanic arcs could reflect along-strike structural and compositional variations (for example, due to the presence of fracture zones) in downgoing subducting plates. For example, Aleutian arc volcanoes (that is, Seguam and Yunaska) situated above the subducted Amlia fracture zone ( Fig. 1 ) are characterized by unusual enrichment of the fluid-mobile element boron [23] , [24] , [25] . High ratios of B/La and B/Be in lavas from this region are attributed to modification of the magma source(s) by unusually high fluxes of aqueous fluids presumably released from serpentine-rich rocks in the downgoing slab. Another example is Mount Shasta, the largest stratovolcano of the Cascades range. The presence of melt inclusions (MIs) with up to nearly 4% H 2 O (ref. 26 ) in unusual high-Mg andesites with elevated Sr/Y and δ 18 O (refs 27 , 28 ), and relatively high volcanic output in this sector of the arc have been attributed to subduction of the Blanco fracture zone beneath this area. Augmented fluid fluxes from fracture zone serpentinites [10] , [29] , [30] could account for enhanced melt productivity and for some of the anomalous geochemical features. Similarly, water-rich magmas from Colima and El Chichon volcanoes in the Trans-Mexican Volcanic Belt [31] , and from Nevado de Longaví (high Ba/Th, Sr/Y and La/Yb ratios [11] , [32] ), Villarrica and Llaima (high U/Th and Pb/Ce ratios [33] ) volcanoes in the Andean Southern Volcanic Zone [11] could reflect locally anomalous fluxes of slab-derived fluids associated with subduction of the Rivera, Tehuantepec [14] , Mocha [11] and Valdivia fracture zones, respectively ( Fig. 1 ). 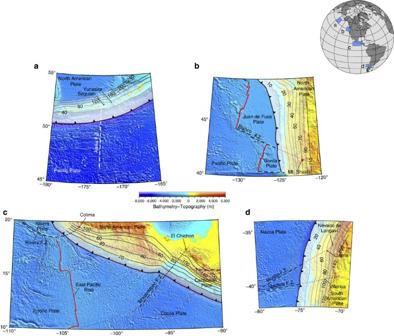Figure 1: Bathymetry and topography maps for four distinct subduction zones. Colour-coded maps (SRTM30_PLUS dataset65) for the (a) Aleutian, (b) Cascadia, (c) Mexican and (d) southern South America subduction zones. The location of fracture major zones is indicated with dashed lines, and volcanic centres characterized by highly hydrated magmas are displayed as red spots. Black isodepths lines show the position of the subducting slabs66,67. FZ, fracture zone. Figure 1: Bathymetry and topography maps for four distinct subduction zones. Colour-coded maps (SRTM30_PLUS dataset [65] ) for the ( a ) Aleutian, ( b ) Cascadia, ( c ) Mexican and ( d ) southern South America subduction zones. The location of fracture major zones is indicated with dashed lines, and volcanic centres characterized by highly hydrated magmas are displayed as red spots. Black isodepths lines show the position of the subducting slabs [66] , [67] . FZ, fracture zone. Full size image Here, we present evidence that anomalous enrichment of B (B/Zr ratio) and other fluid-mobile elements in arc magma sources in several regions strongly correlate with subduction of major fracture zones ( Fig. 1 ), but not in the relatively warm Cascadia and Mexican subduction zones. We infer that fracture zone subduction locally enhances fluid introduction beneath volcanic arcs, but that retention of slab fluids to sub-arc depths depends on subduction zone thermal gradient and approaches negligible efficiency in the warmest subduction zones. We then use three-dimensional high-resolution coupled petrological-thermomechanical numerical models to simulate the physical processes associated with subduction of fracture zones (more details can be found in Methods and Supplementary Table 1 ). The numeric models robustly reveal that partial melts and fluids focus above the slab in areas where fracture zones are subducted. Along-arc geochemical variations To further assess variations in slab-derived fluid inputs to the sub-arc mantle wedge, we consider regional geochemical variations in lavas from the aforementioned volcanic arcs. Unfortunately, direct measurements of water fluxes are poorly constrained in a regional sense owing to relatively sparse measurements of water contents in MIs, as well as the difficulty in relating such measurements directly to slab inputs (see Supplementary Note 1 ). Owing to the high solubility of B in aqueous solutions ( cf. ref. 34 ), this element can serve as a useful proxy for infiltration of slab-derived fluids, and sufficient data are now available for boron contents in arc lavas to evaluate regional patterns in fluid inputs for some arcs. In contrast to intraplate volcanic rocks (for example, mid-ocean ridge or ocean island basalts), arc lavas commonly exhibit selective enrichment of B relative to other highly incompatible elements such as Nb or Zr ( cf. ref. 35 ). Elevated B/Nb or B/Zr ratios in arc lavas can be attributed to inputs to the mantle wedge of aqueous fluids released by devolatilization of subducted materials [36] . Importantly, because all of these elements (B, Zr, Nb, La, Ba and in general all highly incompatible elements) partition similarly into silicate melts ( cf. refs 37 , 38 ), selective enrichment of B in magma sources cannot plausibly be attributed to melt-forming processes or to subsequent magma differentiation processes. Moreover, a slab origin is strongly implicated because B-enrichment in several arcs is strongly correlated with that of 10 Be, which is uniquely added to the mantle via subduction [39] . For convenience, and because high-quality data for Zr are more readily available than for Nb, here we mainly employ the B/Zr ratio as an indicator of relative variations in fluid inputs beneath each of the volcanic arcs considered; this ratio also generally correlates with measured water content in MIs from arc lavas ( cf. Supplementary Fig. 1 and Supplementary Note 1 ). Where available, B/Nb, B/La and similar ratios mimic the trends defined by B/Zr ( Fig. 2 ). Along-strike variations in B-enrichment can be explained by fluctuations in the B inventory of the slab as well as differences in the thermal gradient, hence devolatilization history of the subducting slab. It is likely that these factors are relatively consistent for arc segments where the subducting slab comprises ‘normal’ or uncomplicated oceanic lithosphere of similar age and thermal maturity. Conversely, along-strike variations in B-enrichment (that is, in B/Zr) in a restricted arc segment may either signify differences in source modification, or be attributed to local influences in magmatic processes as will be discussed below. The data considered in this paper are drawn from our own investigations and from published works where available ( cf. Supplementary Note 2 for data sources; cf. Supplementary Note 3 , Supplementary Tables 2–7 and Supplementary Fig. 2 on analytical details, precision and accuracy for new data). The compiled results are shown in Fig. 2 for the southern Andes and the Aleutians, both of which are associated with relatively cool subduction zones, and for the Cascades and the Trans-Mexican volcanic arcs, both of which correspond to young subduction zones with local extensional tectonics. B/Zr ratios are plotted versus along-arc position in latitudinal or longitudinal coordinates, bulk SiO 2 contents and Ba/Zr ratios. It should be noted that most samples are situated near the main volcanic front, albeit the Cascades and Andean data locally include samples ranging from frontal- to back-arc sites. For each arc, effort was made to include primitive mafic lavas but intermediate and evolved compositions are also included to provide better spatial coverage. Most samples are of Quaternary age (<1 Ma). Note that data are also compiled for northern sectors of the Andes, but not discussed in any detail here. Northern Volcanic Zone volcanoes (mostly Ecuador) occur in a region of aseismic ridge subduction that adds considerable complexity to geodynamic considerations. Central Volcanic Zone (CVZ) samples are dominantly silicic (andesite to rhyolite) and too old ( ca. 4 Ma or older age) to reflect modern subduction tectonics; moreover, many of the analyzed samples in this region exhibit evidence of strong crustal influence and are of dubious value in assessing arc mantle processes. In any case, B/Zr values observed in Quaternary age Northern Volcanic Zone and CVZ samples are comparable to those seen in Southern Volcanic Zone (SVZ) samples. 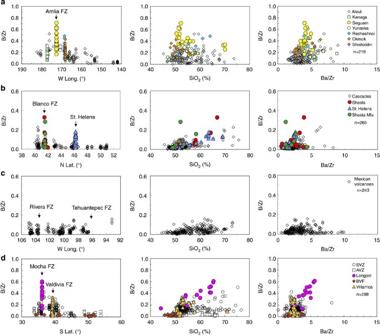Figure 2: Fluid-mobile element geochemistry of selected volcanic arcs. Fluid-mobile element geochemistry shows variation in whole-rock B/Zr as functions of along-strike position and proximity to major fracture zones (FZ), silica content and covariation with Ba/Zr ratios for (a) Aleutians, (b) Cascades, (c) Mexico and (d) Andes volcanic arcs. Most B data were obtained by Prompt Gamma Neutron Activation (see refs24,49) or ICP Emission Spectroscopy (see ref.32) and uncertainties on plotted ratios generally are comparable to symbol size (seeSupplementary Note 3for full analytical details). The number (n) of B/Zr values is shown for each arc; counts for other parameters are given inSupplementary Dataset 1. AVZ, Austral Volcanic Zone (48–55°S); SVZ, Southern Volcanic Zone (33–46°S); BVF, behind volcanic front; MIs, melt inclusions. Figure 2: Fluid-mobile element geochemistry of selected volcanic arcs. Fluid-mobile element geochemistry shows variation in whole-rock B/Zr as functions of along-strike position and proximity to major fracture zones (FZ), silica content and covariation with Ba/Zr ratios for ( a ) Aleutians, ( b ) Cascades, ( c ) Mexico and ( d ) Andes volcanic arcs. Most B data were obtained by Prompt Gamma Neutron Activation (see refs 24 , 49 ) or ICP Emission Spectroscopy (see ref. 32 ) and uncertainties on plotted ratios generally are comparable to symbol size (see Supplementary Note 3 for full analytical details). The number ( n ) of B/Zr values is shown for each arc; counts for other parameters are given in Supplementary Dataset 1 . AVZ, Austral Volcanic Zone (48–55°S); SVZ, Southern Volcanic Zone (33–46°S); BVF, behind volcanic front; MIs, melt inclusions. Full size image B/Zr ratios vary considerably in each of the arcs investigated, but usually exceed typical values (~0.01) for intraplate basalts with exception of some basalts from the Cascades and Mexican arcs. Maximum (and higher median) B/Zr values are seen in lavas from the relatively cool Aleutian and Andean arcs, and lower B/Zr values (some approaching intraplate values) are observed in the warm Cascades and Mexican arcs. This pattern is consistent with more dramatic loss of B and fluids from warmer slabs, and with progressive depletions across arcs as individual slabs become warmer with greater depth ( cf. ref. 40 ). Most notably, along-arc profiles for the Aleutians and southern Andes exhibit conspicuous spikes in B/Zr, where major fracture zones project beneath the arcs (data highlighted in yellow and magenta in Fig. 2 ). The definition of such spikes is somewhat arbitrary, but in the Aleutians B/Zr ratios in Seguam basalts (0.3–0.7) exceed those of nearly all other basaltic lavas in the arc as previously noted [23] , [24] . At Longaví mafic lavas are scarce, but mafic enclaves have higher B/Zr values than seen in proximal SVZ basaltic lavas; additionally, andesitic and dacitic lavas have strikingly higher B/Zr (all >0.3) than their SVZ counterparts, with the exception of basaltic andesites and andesites from Villarrica volcano. We note that these Andean anomalies are specific to Longaví and Villarrica and that samples from surrounding monogenetic mafic volcanoes have relatively low B/Zr values (<0.2) that seem to be representative of the SVZ in general. In contrast, the Cascades and Mexican volcanic arc profiles show only modest B-enrichment overall (B/Zr below 0.15 for most samples, and many below 0.05). In the Cascades, weak ‘spikes’ in B/Zr occur near Mt. Shasta and Mt. St. Helens, albeit basalts from these volcanoes have low B/Zr values characteristic of much of the arc. There are no pronounced spikes evident in the Mexican arc. Data coverage is sparse near the projected locus of the Tehuantepec fracture zone (for example, near El Chichon). Whereas the projected subduction trajectory of the Rivera fracture zone passes beneath the well-sampled Colima Graben region. Subdued B-enrichment in this region could result from unique tectonic conditions (for example, presence of a slab gap beneath Colima [41] ) as well as a higher temperature of the slab subducting under Mexico. To better understand the significance of observed B/Zr spikes, this ratio is also shown as a function of whole-rock SiO 2 content ( Fig. 2 ). Each highlighted case comprises a spectrum of basaltic to dacitic lavas. Notably, elevated but varied B/Zr ratios in the mafic lavas suggest that their mantle sources have been enriched in B, albeit not uniformly so. At Seguam, all basaltic lavas have strongly elevated B/Zr values (approximately 0.3–0.6), and the range is likely inherited from variable fluid (and B) inputs to the mantle source of these lavas. More evolved Seguam lavas have B/Zr ratios overlapping the lower end of the range for basalts from this volcano, and consistent with their derivation by fractional crystallization of such parental magmas. At Longaví, elevated B/Zr ratios (approximately 0.2–0.4) in the most mafic lavas are consistent with source modification exceeding that elsewhere in the Andean SVZ [32] . Even higher B/Zr ratios (up to ~0.6) in the evolved lavas may reflect involvement of more strongly modified sources, fractional crystallization from comparably B-enriched parental magmas (apparently unerupted) or an open-system process whereby B-enrichment is enhanced. Elsewhere in the SVZ, corresponding approximately to the projected locus of the Valdivia fracture zone, basalt to andesite lavas from the sector (lat. 39.4° to 40.5° S) between Villarrica and Puyehue stratovolcanoes also have relatively high B/Zr (0.2–0.3). However, as previously noted, basaltic lavas from monogenetic vents near these volcanoes have lower B/Zr (<0.1), and it appears that B-enrichment in the underlying mantle wedge must be heterogeneous and less extensive than at Longaví. We also note that very high B/Zr values seen in some evolved lavas (SiO 2 >~70%) from the Andean CVZ are not correlated with fracture zone subduction, and likely reflect zircon fractionation or magma interaction with (or derivation from) B-rich lithologies (for example, sediments, evaporates) in the shallow Andean crust [42] , [43] . Basaltic lavas near Mt. Shasta and Mt. St. Helens have B/Zr ratios (approximately 0.02–0.10) only slightly higher than observed in intraplate lavas, and essentially overlapping the range observed for mafic lavas elsewhere in the Cascades arc. Typically, Cascades B/Zr values increase progressively with SiO 2 content, and maximum values rarely exceed ~0.2 (the highest observed value is for a Shasta dacite; ~0.3). Thus, there is little evidence for pronounced B-enrichment anywhere in the Cascades. Published data for Cascades MIs indicate relatively low H 2 O contents (for arcs) typically on the order of 2% or less for basaltic magmas [26] , [44] , [45] , [46] and up to 2–4% in lavas of intermediate and more evolved composition [45] , [47] . As noted earlier, the relatively ‘dry’ character of Cascades volcanic rocks likely reflects strong devolatilization of the young and slowly subducting Cascadia slab, with significant fluid (and B) losses beneath the frontal arc region ( cf. refs 48 , 49 ). MIs from Mt. Shasta area samples typically have low-B contents and B/Zr ratios overlapping values for whole rock lavas ( Fig. 2 ). However, two MIs from a hybrid high-Mg andesite lava (Whaleback shield volcano) do have elevated B and B/Zr (nearly 0.3 in a basaltic andesite glass [45] ), which could be attributed to at least occasional influx of B-rich fluids beneath that region. Because Ba is commonly considered to be a fluid-mobile element, and a proxy for involvement of slab-derived fluids in arc magmas ( cf. ref. 50 ), B/Zr and Ba/Zr ratios are also compared in Fig. 2 . Normalization to Zr emphasizes selective B or Ba fractionation because of processes other than melting or crystal fractionation, neither of which is likely to significantly modify these ratios, except possibly in strongly evolved magmas. Notable separation of Seguam and Longaví lavas from the bulk Aleutian and Andean fields, respectively, emphasizes unique modifications of their sources relative to other sectors of these arcs, and clearly B is the stronger discriminant of the two. In contrast, for the Cascades and Mexico arcs there is significant variation in Ba/Zr with only modest variation in B/Zr, and little evidence for anomalous source modifications along strike. Thus, in relatively dry and hot subduction zones, Ba-enrichment may dominantly reflect input of a sediment melt component, rather than a fluid, as proposed by some authors [51] . Numerical modelling To better understand how subduction of mechanically weak fracture zone rocks may account for unusual arc volcanism ( Fig. 1 ), we use high-resolution three-dimensional coupled petrological-thermomechanical simulations of fracture zone subduction to predict the spatial evolution of melt and hydrous fluid content above subducting slabs in these settings. As detailed in the Methods section, we performed numerical experiments to evaluate the effect of laterally heterogeneous subducting plates by introducing a mechanically weak fracture zone corresponding to a predefined set of plate age offsets and rheological parameters (see Supplementary Fig. 3 ). The rheology of fracture zones is not well known, although it is commonly accepted that they are serpentinized and mechanically weak [9] . Our approach towards evaluating the effect of fracture zone subduction involves a set of numerical models covering initial conditions that range from a simple subduction model with an oceanic plate age offset only, to more complex models incorporating the presence of a weak and partially serpentinized layer corresponding to the location of a fracture zone. 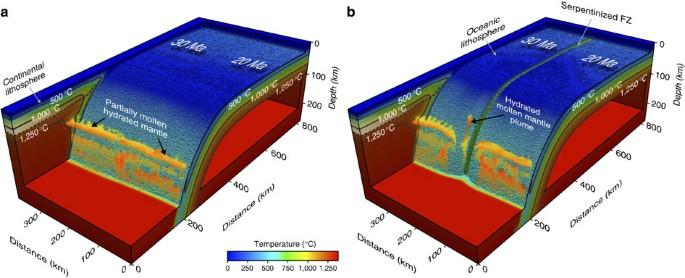Figure 3: Temperature and composition after 17.5 Myr of convergence. (a) Numerical experiment with a heterogeneous subducting plate (20–30 Ma). (b) Numerical experiment with a heterogeneous subducting plate (20–30 Ma) and partially serpentinized fracture zone (hserp. f.z.=10 km;ρserp. f.z.=2,800 kg m−3). Green strip in the middle of the oceanic plate represents the serpentinized fracture zone, and partially molten mantle above the slab is coloured according to the temperature. Dashed line represents the base of the continental lithosphere. Figure 3a shows the result of a subduction experiment after 17.5 Myr of convergence where the oceanic plate includes an age offset of 10 Ma, but without a preexisting lithospheric weakness located across the age offset. During subduction, the progressive hydration of the mantle wedge by slab dehydration induces partial melting above the subducting plate at a depth of ~125 km. The melting front accumulates rather uniformly along strike with no significant variations caused by the presence of the 10 Ma age offset in the oceanic lithosphere ( Fig. 3a ). Also the slab temperature is not affected other than the normal temperature distribution specific for the presence of a 10 Ma age offset ( Fig. 4a ). Similarly uniform melt distributions in the mantle wedge (and slab temperature profiles vs depth) are observed when we increased the lithospheric age shift in the incoming oceanic plate from 5 to 20 Ma ( Supplementary Fig. 4 ) or varied the incoming slab age from 10 to 50 Ma ( Supplementary Fig. 5 ). To evaluate further the impact of fracture zone subduction on arc magma sources along arcs, we added the presence of a mechanically weak zone. For this set of simulations, we impose a narrow (10 km wide) weak zone extending vertically downward from the base of the oceanic crust to a depth of several kilometers into the upper part of the lithosphere. To cover a realistic range of parameters specific for serpentinite rocks associated with fracture zones, we varied the maximum depth (5–10–20 km) and density (2,800–3,000–3,200 kg m −3 ) of the serpentinized layer ( Fig. 2b,d ). Figures 3b and 4b display the result of a subduction experiment after 17.5 Myr of convergence where we include a 10-km wide by a 10-km deep mechanically weak zone, with a rheology specific for serpentinite. In contrast with previous experiments, this model shows several striking features regarding melt distribution in the mantle wedge and slab temperature. The presence of a weak fracture zone in the subducting slab perturbs the uniform distribution of melt in the mantle wedge and triggers the development of an upwelling plume of partially molten and hydrated mantle rocks, locally enhancing the melt productivity in the wedge ( Figs 3b and 4b ). The formation of the upwelling plume starts ~12 Myr after subduction initiation, and then attains its full growth at ~17.5 Myr (see Supplementary Fig. 6 ). The subducting slab temperature distribution is also strongly affected, whereby the weak fracture zone locally increases the temperature at the top of the slab by almost 100 °C ( Fig. 4b ). A closer examination of the subduction process reveals that the weakened serpentinized fracture zone is partially scraped out in the forearc region because of its low strength and positive buoyancy. This in turn creates a trench-orthogonal linear depression on the surface of the slab that subsequently is in-filled by hot surrounding mantle material ( Fig. 5 ). Resulting high temperatures accelerate dehydration of the subducting slab and serpentinite and release of H 2 O-rich fluids above the fracture zone, causing extensive hydration of the overlying ultramafic mantle wedge. In such regions, plume-like instabilities may be triggered by excessive fluxing of hydrous fluids (0.2–0.7-wt% of slab-derived water) released into the mantle wedge by the serpentinized fracture zone, and driven upward at shallower levels by compositional variations, density contrast and viscous heating [52] . We postulate that fluid-mobile trace elements such as B are released in excess as well, owing to their concentration in and release from the serpentinized materials. Because less fluid-mobile elements (for example, Zr, Nb) are less likely to be released in an equally efficient manner, the slab-derived fluids could impose a ‘B-spike’ on infiltrated regions of the mantle wedge while simultaneously facilitating the onset of melting to produce arc magmas. For example, if subduction zone fluids can carry 100’s of p.p.m. B (and essentially no Zr, Nb, La), the amount of fluid required to change B/Zr in primitive mantle (for example, OIB source) to typical modified arc mantle may be only a few tenths of a percent by weight; and to reach higher B/Zr associated with fracture zone subduction, only slightly higher proportions of fluid are required ( cf. ref. 53 ). Figure 3: Temperature and composition after 17.5 Myr of convergence. ( a ) Numerical experiment with a heterogeneous subducting plate (20–30 Ma). ( b ) Numerical experiment with a heterogeneous subducting plate (20–30 Ma) and partially serpentinized fracture zone ( h serp. f.z. =10 km; ρ serp. f.z. =2,800 kg m −3 ). Green strip in the middle of the oceanic plate represents the serpentinized fracture zone, and partially molten mantle above the slab is coloured according to the temperature. Dashed line represents the base of the continental lithosphere. 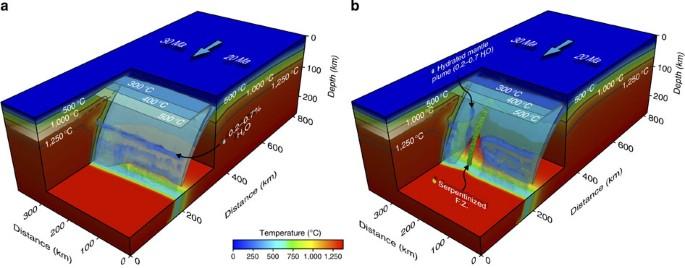Figure 4: Slab temperature and H2O distribution after 17.5 Myr of convergence. (a) Numerical experiment with a heterogeneous subducting plate (20–30 Ma). (b) Numerical experiment with a heterogeneous subducting plate (20–30 Ma) and partially serpentinized fracture zone (hserp. f.z.=10 km;ρserp. f.z.=2,800 kg m−3). Slab temperature is shown as semitransparent (blue tones) isosurfaces and hydrated mantle and plume above the slab is coloured in light blue. Full size image Figure 4: Slab temperature and H 2 O distribution after 17.5 Myr of convergence. ( a ) Numerical experiment with a heterogeneous subducting plate (20–30 Ma). ( b ) Numerical experiment with a heterogeneous subducting plate (20–30 Ma) and partially serpentinized fracture zone ( h serp. f.z. =10 km; ρ serp. f.z. =2,800 kg m −3 ). Slab temperature is shown as semitransparent (blue tones) isosurfaces and hydrated mantle and plume above the slab is coloured in light blue. 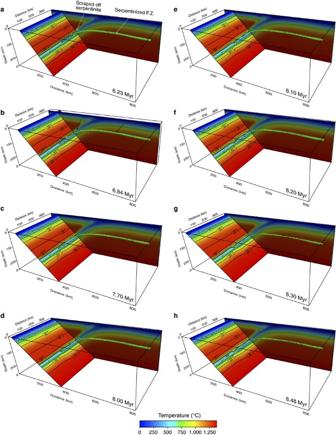Figure 5: Slab temperature evolution for a subduction experiment with serpentinized fracture zone. (a–h) The evolution from 6.23 to 8.48 Myr. The partially serpentinized fracture zone has the following characteristics:hserp. f.z.=10 km andρserp. f.z.=2,800 kg m−3. The slice through this model is normal to the slab surface and illustrates that at B8.10 Myr the slab temperature starts to increase in the region of fracture zone subduction (e). Full size image Figure 5: Slab temperature evolution for a subduction experiment with serpentinized fracture zone. ( a – h ) The evolution from 6.23 to 8.48 Myr. The partially serpentinized fracture zone has the following characteristics: h serp. f.z. =10 km and ρ serp. f.z. =2,800 kg m −3 . The slice through this model is normal to the slab surface and illustrates that at B8.10 Myr the slab temperature starts to increase in the region of fracture zone subduction ( e ). Full size image There is strong evidence for anomalous enrichment of B and other fluid-mobile elements in arc magma sources associated with subduction of fracture zones ( Figs 1 and 2 ). This is best explained in terms of infiltration of anomalous volumes of B-rich fluids, unusually high B contents in such fluids, or both. To a large degree, this is likely to be a near instantaneous phenomenon (that is, associated with Quaternary subduction rather than a time-integrated effect) because in most cases the locus of fracture zones-arc convergence migrates along the arc with time. The Andes SVZ may be a good place to explore such ‘migratory effects’, because B data there show a broad B/Zr anomaly that may result from such an effect. Although the present data set is too limited to rigorously evaluate spatial-temporal variations in slab fluid proxies, this would be an interesting research topic to pursue in the future. The magnitude of fluid flux to the mantle wedge can only be estimated in a relative sense without more detailed knowledge of actual slab geochemical inventories and consideration of thermal evolution, both of which vary from arc to arc. As previously noted, initial inventories of fluids and fluid-mobile elements in subducting slabs are controlled by geologic factors (for example, degree of alteration of ocean crust, type and thickness of overlying sediments). The presence of fracture zones will likely enhance the initial inventories, but to varying extent judging from differences in B-enrichment associated with the Mocha and Valdivia fracture zones. Retention of these inventories to sub-arc depths hinges on the thermal maturity and metamorphic history of the slab, and is most efficient for cooler slabs. Compared with other arcs, the overall limited B-enrichments in Cascades and Mexican arc lavas can be attributed largely to the advanced thermal maturity of their respective slabs, with significant decimation of initial B inventories before reaching sub-arc depths. In addition, local extension in the Cascades and Mexican arcs may be associated with decompression melting of upwelling asthenospheric mantle that has been little-modified by slab-derived fluids, and produces ‘intra-plate-like’ mafic magmas ( cf. refs 54 , 55 , 56 ). Tectonic imperfections in the subducting slab, such as a postulated slab gap beneath the Colima region in western Mexico [41] , could also allow upwelling of asthenospheric mantle. In some instances, large variations in B/Zr (and similar ratios) are observed at individual arc volcanoes or local regions. Among many possibilities, a likely explanation is that the mantle wedge is heterogeneously modified by slab inputs. In cool subduction zones, high fluid flux may overwhelmingly modify the mantle wedge; conversely, in warm subduction zones with low fluid flux, the mantle wedge may be modified only slightly (or locally). In the latter case (for example, Cascades or Mexico), a greater diversity of magma types is seen, some of which may be derived from hardly modified asthenospheric mantle. Finally, as illustrated in Supplementary Note 1 , trace element proxies for fluxes of slab-derived fluids in subduction zones are imperfect, as are direct estimates of magmatic fluid contents. The proxies are best used to assess relative differences in slab fluid fluxes within individual volcanic arcs where physical subduction parameters (plate age, subduction rate) are comparable along strike. Critical to our understanding of arc magma genesis and its along-arc variability is the melting zone distribution in the mantle wedge above the subducted fracture zone. To illustrate how fracture zones influence melt patterns above slabs, we employed three-dimensional high-resolution coupled petrological-thermomechanical numerical models of subduction. Modelling results show that pure thermal gradients across fracture zones in the oceanic slabs are not able to explain the observed anomalous enrichment in fluid-mobile elements in arc magma sources associated with subduction of fracture zones ( Fig. 3a ). However, introducing a zone of weakness corresponding to the position of fracture zone, our modelling suggests that regional variations of both slab temperature and mantle wedge melt distribution are guided by the position of the subducted fracture zone ( Figs 3b and 4b ). The combination of low strength and positive buoyancy (partial serpentinization) associated with a fracture zone produces a trench-orthogonal linear depression on the surface of the slab that is in-filled by hot surrounding mantle material ( Supplementary Fig. 6 ). The increased slab temperature in this region causes a stronger dehydration of the incoming plate along the fracture zone, triggering a partially molten and hydrated thermal-chemical instability ( Supplementary Fig. 6 ). Considering a wide range of parameters related with the fracture zone (densities of 2,800–3,200 kg m −3 , and thicknesses of 5–20 km), our modelling predicts consistent outcomes: that is, the numerical results show the same pattern for mantle wedge melt/fluid distribution along the strike and the development of partially molten hydrous instabilities above the subducted serpentinized fracture zone ( Supplementary Fig. 7 ). Our modelling results are in good agreement with recent studies in the Villarrica region of the Andean SVZ that revealed the existence of physical anomalies related to the subduction of the Valdivia fracture zone ( Fig. 1 ). Specifically, the projected trace of this fracture zone, between 39°S and 40°S in the forearc region, corresponds to a negative gravity anomaly of −50 mGal (refs 57 , 58 ), a local minimum in plate coupling and aseismic slip [59] , and reduced seismic velocities coupled with an increased V p / V s ratio [33] , all of which suggest the localized existence low-strength/low-density material and enhanced fluid release. In this study, combined geochemical observations and robust numeric modelling results confirm that the subduction of weak serpentinized fracture zones is a first-order geodynamic process that contributes to significant variations in the composition and fluid content of magmas along volcanic arcs. Model parameters and boundary conditions The modelling was performed using the finite difference code I3ELVIS with marker-in-cell technique and multigrid approach [60] . The three-dimensional numerical model simulates self-sustaining subduction of an oceanic plate beneath a continental plate, where only internal forces drive the model evolution. The computations are performed within a Cartesian domain 808 km long, 392 km wide and 264 km deep ( Supplementary Fig. 3 ). This domain is evenly divided into 404 × 196 × 132 Eulerian grid cells (corresponding to a 2 × 2 × 2 km staggered grid resolution), which contain 180 million randomly distributed Lagrangian markers. The mechanical boundary conditions are as follows: the top boundary is free slip and the bottom boundary is permeable in the vertical direction; lateral boundaries are free slip except the lateral boundary corresponding to the oceanic plate, which has prescribed a constant subduction velocity of 6.5 cm per year, and the lateral boundary corresponding to the oceanic plate, which has a non-slip condition. The subducted oceanic crust includes an upper layer of sediments (2 km thick) overlying a 2-km thick layer of basalt and a 5-km thick layer of gabbroic rocks. The continental crust comprises an upper layer (23 km thick) and a lower layer (12 km thick) of felsic rocks. The mantle consists of anhydrous peridotite (see material properties in Supplementary Table 1 ). The initiation of subduction is set by introducing an initial rheological weak zone with wet olivine rheology and low brittle/plastic strength ( Supplementary Fig. 3b ). The top surface of the model is treated as an internal free surface by using a 12-km thick top layer with low viscosity and low density (10 18 Pa s and 1 kg m −3 ), overlying a 3-km thick water layer (10 18 Pa s and 1,000 kg m −3 ). This weak layer is used to minimize shear stresses (<10 4 Pa) and reproduce free surface at the top of the lithosphere [61] . The initial thermal structure is described by a thermal boundary layer (age controlled) at the top (see Supplementary Fig. 3a ). The initial fracture zone geometry corresponds to the location of the ocean plate age offset. In our models, water is present in sediments, hydrothermally altered basalt and serpentinized fracture zone. Slab dehydration and mantle hydration reactions are assigned for P-T conditions computed from the thermodynamic database. Proportion of serpentine in hydrated mantle is limited by the 2 wt% cutoff limit of water content because of assumed incomplete (large-scale) serpentinization, which is in agreement with seismic constraints [17] , [62] . In addition, latent heat of partial melting and crystallization is taken into account. We use fluid markers to show the release and propagation of fluids into the overlying mantle wedge. Dehydration reactions lead to the release of a certain amount of fluid that is stored in a water marker. We imposed an upward vertical speed for free water of 10 cm per year. When this water marker encounters a rock capable of absorbing water, either by hydration or melting reactions, the fluid marker is consumed [63] . Rock markers are used to compute equilibrium water content at each numerical time step with the help of P-T-H 2 O tables computed with PERPLE_X [63] . We also included markers in the modelling of melting processes where both, hydrous and dry melting, are a nonlinear function of pressure and temperature [64] . Markers track the amount of melt extracted, and the total amount of melt for every marker takes into account the amount of previously extracted melt. We use a constant viscosity of 10 19 Pa s for partially molten rocks in all our numerical experiments, and the lower and upper cutoff range for viscosity of all types of rocks is 10 19 –10 24 Pa s. Other parameters used in the numerical model are shown in Supplementary Table 1 . How to cite this article: Manea, V. C. et al. Subduction of fracture zones controls mantle melting and geochemical signature above slabs. Nat. Commun. 5:5095 doi: 10.1038/ncomms6095 (2014).